Regioselective radical α-borylation of α,β-unsaturated carbonyl compounds for direct synthesis of α-borylcarbonyl molecules Organoboron compounds are highly valuable in synthetic chemistry. In particular, α-borylcarbonyl compounds have shown versatile synthetic applications, owing to fruitful chemistries of both the boryl and carbonyl moieties. However, the synthesis of these molecules still remains tedious and time-consuming. Here we report a straightforward and practical route to synthesize α -borylcarbonyl molecules based on a regioselective radical α -borylation of α , β -unsaturated carbonyl compounds. The reaction features unusual α -regioselectivity and high functional-group compatibility. Further synthetic applications of new α -borylated products were also demonstrated. DFT and kinetic studies implicated that the α -regioselectivity of β -aryl- α , β -unsaturated carbonyl compounds was determined by the thermodynamically more favorable radical α -addition step, whereas the formation of α -addition products from β -alkyl- α , β -unsaturated carbonyl compounds was driven by an energetically favored hydrogen atom transfer step. Given that α , β -unsaturated carbonyl compounds can be easily obtained in abundance and variety, this method enjoys great advantages in diverse and economical synthesis of valuable α -borylcarbonyl molecules. Organoboron compounds have been substantially applied in chemical synthesis, medicinal chemistry, and material sciences [1] . Borylative functionalization of alkenes is among the most widely used methods to access these products [2] , [3] , [4] , [5] , [6] . In this context, great endeavors have been devoted to exploit borylation reactions of α , β -unsaturated carbonyl compounds, owing to their easy accessibility and intrinsically high electrophilicity. Over the past decades, many reagents and conditions have been well established to synthesize β -borylcarbonyl compounds through nucleophilic β -borylation [7] , [8] , [9] , [10] . In sharp contrast, the direct α -borylation reaction to access isolable α -borylcarbonyl molecules remains a formidable challenge [11] , mainly because the products undergo facile 1,3-boron shift to give thermodynamically more stable O-boron enolates [12] . Thus, developing practical and broadly applicable new α -borylation methods that can make stable and structurally diverse α -borylcarbonyl compounds is highly desirable. α-Borylcarbonyl compounds with the boron center being quaternized by a Lewis base are air stable and easily handled [13] , [14] , [15] . In these molecules, both the boron and carbonyl moieties can be manipulated to install various functionalities of interest. This strategy has shown important applications in a variety of research fields and thus the synthesis of stable α-borylcarbonyl compounds has captured considerable attention in synthetic chemistry [13] , [14] , [15] , [16] , [17] , [18] , [19] , [20] . For example, He and Yudin [21] , and Li and Burke [22] independently reported the synthesis of amphoteric α-boryl aldehydes from oxiranyl boronates by a Lewis acid-promoted 1,2-boryl migration (Fig. 1a ). Wang and colleagues [23] , and Yudin and colleagues [24] have developed oxidative functionalization reactions of alkenylboronates to make α -boryl ketones (Fig. 1b ). In addition, Curran and colleagues [25] , [26] , Zhou and colleagues [27] , [28] , [29] , Xu and colleagues [30] , and Arnold and colleagues [31] have described a number of catalytic B−H insertion reactions of Lewis base-boranes and α -diazocarbonyl compounds (Fig. 1c ). Despite these advances, the preparation of these starting materials usually required multi-step synthesis, which limits the functionality and applicability. Various structurally diverse α , β -unsaturated carbonyl compounds are readily accessible. Arguably, the direct α -borylation of α , β -unsaturated carbonyl compounds to access value-added α -borylcarbonyl molecules is a more straightforward and economical strategy. However, this has rarely been documented. During the reviewing of this manuscript, Ingleson and colleagues [32] reported an iodine-catalyzed ionic hydroboration of α , β -unsaturated esters. Herein, we report a conceptually distinct regioselective radical α -borylation protocol by taking advantages of the chemical reactivity of N -heterocyclic carbene (NHC)−boryl radical (Fig. 1d ). Using radical cascade strategy, complex boron-substituted cyclic frameworks can be constructed as well. Fig. 1 Synthesis of stable α-borylcarbonyl molecules. a Lewis acid-catalyzed 1,2-boryl migration of oxiranyl boronates. b Oxidative functionalization of borylated alkenes. c B−H Insertion reactions of Lewis base-boranes and α-diazocarbonyl compounds. d This work: radical α-borylation of α , β -unsaturated carbonyl compounds Full size image Reaction design Recent years have witnessed the significant progress in NHC−boryl radical chemistry [33] , [34] , [35] , [36] , [37] , [38] , [39] , [40] , as the pioneering work of Curran and colleagues [41] . Our group has been interested in the exploration of new radical borylation methods to create C−B bonds from alkenes and alkynes [42] , [43] . Our previous studies revealed that the NHC−boryl radical addition to alkenes should be a reversible process and the reaction equilibrium is favored to the addition products when the resulted alkyl radicals are stabilized by an adjacent aryl or carbonyl group. In order to get more details of such reactivity, we intended to study the reaction with β -aryl- α , β -unsaturated carbonyl compounds. In this case, competitive α - and β -additions were envisioned to occur and the regioselectivity outcome would give us insightful information to rationalize the reaction profiles. This would further lead to the development of new radical borylation methods. Optimization of reaction conditions We commenced our study by examining the radical hydroboration of ethyl cinnamate ( 1a ) with 1,3-dimethylimidazol-2-ylidene borane (NHC−BH 3 , 2 ) as the boryl radical precursor. Initially, β -addition was assumed to take place preferentially, owing to the strong inductive effect of the carbonyl group and the nucleophilic character of the NHC−boryl radical [44] , [45] , [46] , [47] , [48] . 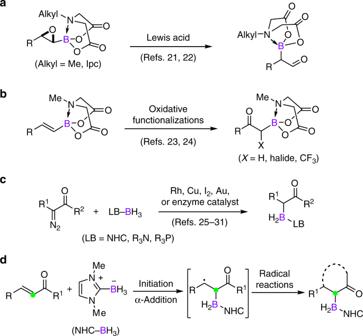Fig. 1 Synthesis of stable α-borylcarbonyl molecules.aLewis acid-catalyzed 1,2-boryl migration of oxiranyl boronates.bOxidative functionalization of borylated alkenes.cB−H Insertion reactions of Lewis base-boranes and α-diazocarbonyl compounds.dThis work: radical α-borylation ofα,β-unsaturated carbonyl compounds Unexpectedly, the reaction only gave α -borylated product 3a in 49% yield in the presence of tert -dodecanethiol as a polarity reversal catalyst [45] (Table 1 , entry 1). The β -addition product was not detected at all. Such a specific α -regioselectivity has rarely been achieved in radical reaction of α , β -unsaturated carbonyl compounds, wherein β -regioselectivity usually predominated [49] , [50] . More importantly, this α -borylation reaction would offer a more straightforward and practical strategy to access valuable α -borylcarbonyl compounds from readily available starting materials. Thus, we decided to study the reaction further. Table 1 Optimization of reaction conditions Full size table The effect of the thiol catalyst was first studied. Increasing the loading of tert -dodecanethiol to 50 mol% gave 3a in an 81% isolated yield (entry 2). Using other thiol catalyst, such as benzenethiols (PhSH, 4-MeOC 6 H 4 SH, 4-CO 2 MeC 6 H 4 SH) and methyl thioglycolate (MeO 2 CCH 2 SH) as the catalyst also led to 3a in comparable yields (entries 3–6). A range of Lewis base−BH 3 complexes were tested as the boryl radical precursors. It was found that NHC−BH 3 complexes, even including an electrophilic boryl radical precursor ( 2d ) [51] could participate in this radical hydroboration, producing the corresponding hydroboration products in good yields (entries 7–9). However, the use of pyridine−BH 3 ( 2e ) and Me 3 N−BH 3 ( 2 f ) could not induce the desired boryl radical addition reaction and 1a was fully recovered (entries 10 and 11). When the reaction was conducted without a thiol catalyst (entry 12), product 3a was not detected, which suggested that the hydrogen atom transfer step might play an important role to control the reactivity and regioselectivity. Moderate yields of 3a were obtained when di- tert -butyl hyponitrite was utilized as the radical initiator (entries 13 and 14). No reaction occurred in the absence of a radical initiator, indicating a radical mechanism is involved in this process (entries 15 and 16). 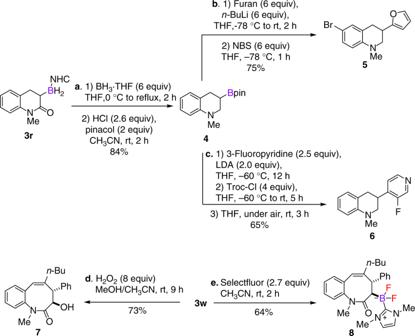Fig. 2 Diversification ofα-borylcarbonyl compounds.aSynthesis of 3-boron-substituted tetrahydroquinoline4via a one-pot transformation from3r.bSynthesis of 3-furan-substituted tetrahydroquinoline5.c. Synthesis of 3-pyridine-substituted tetrahydroquinoline6.dSynthesis ofα-hydroxy product7by the direct oxidation of the boron moiety.eSynthesis of NHC−difluoroboranes8from3w Substrate scope of radical α-borylation reactions The scope and generality of this α -borylation protocol was investigated (Table 2 ). A wide range of α , β -unsaturated carbonyl compounds were converted to α -boryl- β -aryl esters with aryl rings bearing a variety of functional groups (for 3a – 3g ). The presence of additional simple alkene and alkyne motifs did not retard the desired borylation reaction (for 3h – 3j ). Moreover, the intramolecular 6- exo cyclization of the resulted alkyl radicals with an alkyne or alkene tether did not occur for 1,6-enyne 1 h and 1,6-diene 1j , probably due to a slower cyclization step than the hydrogen atom abstraction reaction. A range of β -heteroaryl rings, including indole (for 3k ), quinoline (for 3 l ), and furan (for 3 m ), could be installed. α-Borylation of cumarin proceeded to give the desired product 3n in 72% yield. A mixture of diastereomers (for 3o ) was obtained for the reaction of 1o . Increasing the steric congestion at the α -carbon (for 1p ) led to both α - and β -additions, affording 3p- α and 3p- β in 22% and 53% yields, respectively. The present method allowed for the construction of a series of α -borylated amides (for 3q – 3t ). A gram scale synthesis of 3r was also achieved in 79% yield. The reaction with amide 1t bearing a chiral oxazolidinone unit gave product 3t in a good yield but with low diastereoselectivity. When Lewis acids such as La(OTf) 3 , Zn(OTf) 2 , and MgBr 2 were added to promote the diastereoselectivity [52] , [53] , the desired hydroboration product 3t was not detected and hydrogenation of 1t occurred instead (see Supplementary Table 1 ). Interestingly, the reaction of amide-bridged 1,6-enyne 1 u and 1,6-diene 1 v , both radical hydroboration and radical borylation/cyclization cascades proceeded, whereas the attempts to increase the yield of cyclized products 3 u’ and 3 v’ have been thus far proven unsuccessful. Remarkably, an intriguing 8- endo cyclization [54] , [55] of intermediate A derived from α -borylation of N -( o -ethynylaryl)cinnamamides 1 proceeded smoothly to furnish boron-handled benzazocines (for 3w – 3aa ). Notably, this protocol was also effective for the assembly of α -boryl ketones (for 3ab – 3ad ) and even acid (for 3ae ). As for a limitation, the reaction of cinnamaldehyde resulted in a facile hydride reduction to give the corresponding alcohol and no hydroboration product was observed. 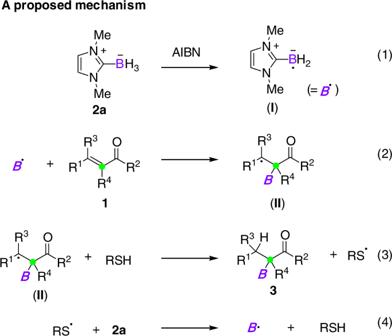Fig. 3 Mechanism. A proposed radical chain process for hydroboration of1 Table 2 Scope of radical α -borylation of β -aryl- α , β -unsaturated carbonyl compounds Full size table Table 3 Scope of radical α -borylation of β -alkyl- α , β -unsaturated carbonyl compounds Full size table The presence of a β -aryl group that can stabilize the resulting alkyl radical intermediates was envisioned to account for the above α -addition selectivity. Based on this assumption, we next turned our attention to study the reaction with β -alkyl- α , β -unsaturated carbonyl compounds (Table 3 ). The lack of aryl resonance stabilization would render the β -addition favorable. 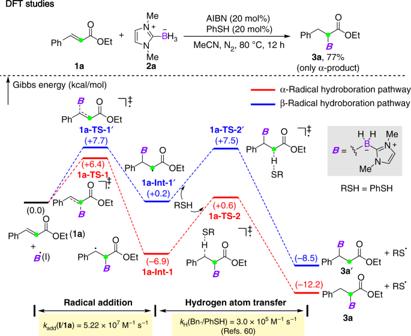Fig. 4 Theoretical calculations. DFT calculations of the radical hydroborylation of1a Surprisingly, when ethyl crotonate ( 1af ) was subjected to the reaction conditions, α -borylation continued to be the major reaction pathway, giving 3af- α in a 41% yield with 26% yield of the β -addition product 3af- β . When PhSH was used as the catalyst, 3af- α and 3af- β were formed in 22% and 45% yields, respectively. The reaction of crotonamide 1ag resulted in superior α -selectivity, albeit with moderate yield. Notably, the introduction of a cyclopropane ring at the β- carbon (for 1ah ) led to only α -addition product 3ah , which was probably driven by the facile ring-opening process. Furthermore, increasing the steric effect on the β -carbon gave solely α -borylated products (for 3ai – 3al ). However, the reaction of ethyl acrylate under the optimized reaction conditions led to polymerization. Synthetic applications of α-borylcarbonyl compounds The conversion of α -borylcarbonyl compounds to various functionalized borylated products have been well studied [13] , [14] , [15] . The present method allowed for the construction of a series of structurally new α -borylated molecules. The synthetic utility of some typical examples was demonstrated (Fig. 2 ). Reduction of the amide moiety of 3r with BH 3 •THF afforded NHC−borane-substituted tetrahydroquinoline, which could be further converted to versatile pinacol boronic ester 4 . The subsequent coupling reactions with heteroaromatic compounds following Aggarwal’s protocols [56] , [57] delivered furan- and pyridine-substituted tetrahydroquinolines 5 and 6 , respectively. In addition, the newly formed boron-handled benzazocines could be transformed to more useful building blocks. For example, oxidation of 3w afforded α -hydroxy product 7 in 73% yield. Treatment of 3w with Selectfluor furnished NHC−difluoroboranes 8 [58] , which represents a new class of stable α -borylcarbonyl molecules that may find potential synthetic applications. Fig. 2 Diversification of α -borylcarbonyl compounds. a Synthesis of 3-boron-substituted tetrahydroquinoline 4 via a one-pot transformation from 3r . b Synthesis of 3-furan-substituted tetrahydroquinoline 5 . c . Synthesis of 3-pyridine-substituted tetrahydroquinoline 6 . d Synthesis of α -hydroxy product 7 by the direct oxidation of the boron moiety. e Synthesis of NHC−difluoroboranes 8 from 3w Full size image Based on the results obtained in this work and previous findings on NHC-boryl radicals [35] , a possible radical chain process was proposed for the hydroboration of α , β -unsaturated carbonyl compounds. As illustrated in Fig. 3 , NHC-boryl radical ( I ) is first generated in the presence of AIBN as the radical initiator. After that, I undergoes addition to the α -carbon of 1 , giving alkyl radical intermediates II . The following hydrogen atom transfer from a thiol catalyst provides hydroboration products 3 . The resulting sulfur radical further abstracts a hydrogen atom from 2a to regenerate I and RSH, thus propagating the radical chain process [45] . Fig. 3 Mechanism. A proposed radical chain process for hydroboration of 1 Full size image In this radical hydroboration process, an unusual α -regioselectivity was observed. To gain more insight into this selectivity, computational and kinetic studies were then performed. For the reaction of 1a , as shown in Fig. 4 , the Density Functional Theory (DFT) studies revealed that the energy barriers of α - and β -additions are comparable (+6.4 kcal mol −1 for α -addition and +7.7 kcal mol −1 for β -addition), while the resulting radical intermediates have significant energy difference (−6.9 kcal mol −1 for 1a-Int-1 and +0.2 kcal mol − 1 for 1a-Int-1’ ). This is probably attributed to more stabilization from the phenyl group than that from the ethoxycarbonyl motif [59] . The subsequent hydrogen atom transfer from the thiol catalyst to 1a-Int-1 and 1a-Int-1’ requires an almost same energy barrier (+7.5 kcal mol −1 for 1a-Int-1 and +7.3 kcal mol −1 for 1a-Int-1’ ). Such a barrier renders the β -addition/elimination step reversible, thus accumulating the thermodynamically more favorable α -addition product 3a . We next used laser flash photolysis (LFP) experiments [44] to measure the rate constant for the addition reaction of NHC-boryl radical ( I ) to 1a . 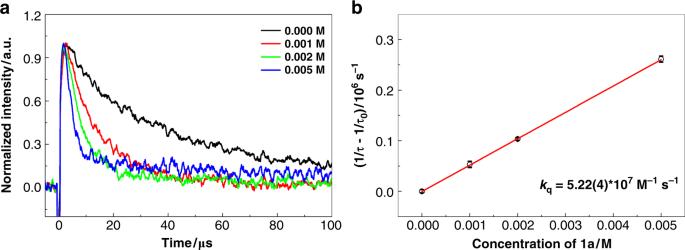Fig. 5 Kinetic studies.aDecay ofIat 400 nm at 25 °C with increasing concentrations of1afrom 0 M to 0.005 M.bStern−Volmer plots generated from the fitted lifetime ofIin the presence of1ain different concentrations at 25 °C 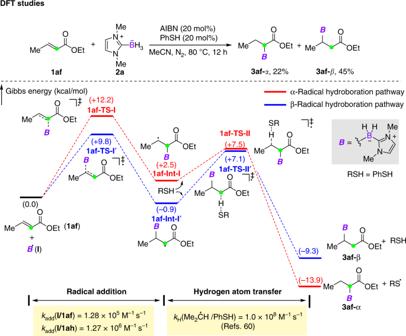Fig. 6 Theoretical calculations. DFT calculations of radical hydroborylation of1af Figure 5a shows the decay curves of absorption of I at 400 nm with increasing concentration of 1a . The bimolecular reaction rate constant k add = 5.22 × 10 7 M −1 s −1 was determined by linear fitting the relationship between the reciprocal of the lifetime of I and the concentration of 1a with the Stern–Volmer equation (Fig. 5b ). It has been reported that the rate constant of hydrogen atom transfer from PhSH to a benzyl radical ( k H ) is 3.0 × 10 5 M −1 s −1 [60] , which is slower than the first radical addition step. Furthermore, the activation parameters ΔH ≠ (−0.180 kcal mol −1 ) and ΔS ≠ (−99.7 J mol −1 ) for the addition to 1a were also determined, thereby giving the Gibbs free energy Δ G ≠ = 6.92 kcal mol −1 (see Supplementary Fig. 11 ). This is comparable with the computational result. Fig. 4 Theoretical calculations. DFT calculations of the radical hydroborylation of 1a Full size image Fig. 5 Kinetic studies. a Decay of I at 400 nm at 25 °C with increasing concentrations of 1a from 0 M to 0.005 M. b Stern−Volmer plots generated from the fitted lifetime of I in the presence of 1a in different concentrations at 25 °C Full size image The reaction of 1af gave a mixture of α - and β -addition products. It should be mentioned that the formation of α -product was quite unusual, because the α -addition intermediate has no β -aryl stabilization. To rationalize such reactivity, a computational study was performed. The free-energy profiles of the reaction between 1af and NHC-boryl radical using PhSH as the catalyst are shown in Fig. 6 . Indeed, in this reaction, the addition of NHC-boryl radical to the α -position of 1af requires a higher activation energy (+12.2 kcal mol −1 ) than that to the β -carbon (+9.8 kcal mol −1 ). Moreover, the resulting α -addition intermediate 1af-Int-I (+2.5 kcal mol −1 ) has higher energy than β -addition intermediate 1af-Int-I’ (−0.9 kcal mol −1 ). However, the subsequent hydrogen atom transfer step to 1af-Int-I undergoes easily with a facile energy barrier of 5.0 kcal mol −1 ( 1af-Int-I → 1af-TS-II ) and an obvious energy decrease of 16.4 kcal mol −1 ( 1af-Int-I → 3af-α ). Such an energetically highly favorable hydrogen atom transfer process renders the α -addition step irreversible. On the other hand, a higher energy barrier of  8.0 kcal mol −1 ( 1af-Int-I’ → 1af-TS-II’ ) is required in the hydrogen atom transfer step because of the unmatched polarity. This calculation suggests that both α - and β -addition products are possible to form and the formation of α -addition product ( 3af- α ) is driven by the thermodynamically and kinetically more favorable hydrogen atom transfer step. The LFP experiments were carried out for the reaction of NHC-boryl radical ( I ) and 1af (see Supplementary Fig. 4 ), giving the apparent rate constant k add = 1.28 × 10 5 M −1 s −1 . As reported, the hydrogen atom transfer from PhSH to the isopropyl radical is very fast (1.0 × 10 8 M −1 s −1 ). Therefore, it is obvious that the radical addition is much slower than that of hydrogen atom transfer step, which is in good agreement with the DFT studies. In addition, as mentioned above, the reaction of 1ah bearing a β -cyclopropane moiety only gave α -addition product. The rate constant for radical addition to this substrate was also measured. As a result, a faster reaction (1.27 × 10 6 M −1 s −1 , see Supplementary Fig. 5 ) as compared with 1af was observed. This suggests that the following facile cyclopropane ring-opening process (1.3 × 10 8 s −1 ) [61] may play a role to facilitate the α -addition. Fig. 6 Theoretical calculations. DFT calculations of radical hydroborylation of 1af Full size image The reaction of 1ai , which has increased steric effect at the β -carbon, only provided α -addition product 3ai . The computational study of this reaction shows that both the activation energies for α - and β -additions, and the energies of the resulting alkyl intermediates are similar (the free-energy profiles are shown in Supplementary Fig. 1 ). However, the following hydrogen atom transfer is energetically more favorable to the α -addition intermediate (+2.4 kcal mol −1 ) than to the β -addition intermediate (+7.3 kcal mol −1 ), thus leading to exclusive α -regioselectivity. The observed rate constant for this radical addition is 4.2 × 10 4 M −1 s −1 (see Supplementary Fig. 6 ), which is much slower than the hydrogen atom transfer from PhSH to a tertiary alkyl radical (1.4 × 10 8 M −1 s −1 ). Overall, the kinetic studies and computational results agree nicely. In summary, we have developed a regioselective radical α -borylation of α , β -unsaturated carbonyl compounds. This method enables a general and practical synthesis of a wide range of valuable α -boryl esters, amides, ketones, and acids from readily available starting materials. This radical α -addition has been rarely achieved for α , β -unsaturated carbonyl compounds, especially for β -alkyl substituted ones. DFT calculations and kinetic studies have been performed to rationalize such regioselectivity. The results indicate that the thermodynamically more favorable α -addition step is responsible for the specific α -selectivity in β -aryl- α , β -unsaturated carbonyl compounds, and an energetically favored hydrogen atom transfer step accounts for the formation of α -borylated products from β -alky -α , β -unsaturated carbonyl compounds. The resulted α -borylated products will have potential applications in synthetic and medicinal chemistry. Exploration of the enantioselective radical α -borylation reactions is currently ongoing in our lab. Radical α -borylation of α , β -unsaturated carbonyl compounds To a 25 ml flame-dried Schlenk flask under nitrogen, NHC-BH 3 ( 2 , 0.500 mmol), substrate 1 (0.600 mmol), AIBN (0.100 mmol), tert- dodecanethiol (0.250 mmol), and CH 3 CN (5 ml) were added. The mixture was stirred at 80 °C for 12 h under nitrogen atmosphere. After evaporation of solvent, the resulting crude material was purified by flash column chromatography (silica gel; petroleum ether/ethyl acetate) to give the corresponding product. Computational methods All the calculations were employed at B3LYP level of theory with an empirical dispersion term (Grimme-D3) as implemented in Gaussian 16 software packages. Geometry optimization was carried out with the 6–31 + G(d) basis set in acetonitrile solvent (using  Solvation Model based on Density). Frequency analysis was calculated at the same level of theory to verify the nature of stationary points. For each transition state, the intrinsic reaction coordinate analysis was conducted to ensure that it connects the right reactant and product. To obtain more accurate energies, single-point energy calculations were performed on all optimized structures applying the 6–311 + G(d, p) basis set. Standard state concentrations of 18.9 and 1.0 mol l −1 were used for MeCN and all the other species, respectively (see Supplementary References 18–25).